Multichannel cavity optomechanics for all-optical amplification of radio frequency signals Optomechanical phenomena in photonic devices provide a new means of light–light interaction mediated by optical force actuated mechanical motion. In cavity optomechanics, this interaction can be enhanced significantly to achieve strong interaction between optical signals in chip-scale systems, enabling all-optical signal processing without resorting to electro-optical conversion or nonlinear materials. However, current implementation of cavity optomechanics achieves both excitation and detection only in a narrow band at the cavity resonance. This bandwidth limitation would hinder the prospect of integrating cavity optomechanical devices in broadband photonic systems. Here we demonstrate a new configuration of cavity optomechanics that includes two separate optical channels and allows broadband readout of optomechanical effects. The optomechanical interaction achieved in this device can induce strong but controllable nonlinear effects, which can completely dominate the device's intrinsic mechanical properties. Utilizing the device's strong optomechanical interaction and its multichannel configuration, we further demonstrate all-optical, wavelength-multiplexed amplification of radio-frequency signals. In nanoscale photonic devices, one optical signal can generate sufficient optical force to mechanically displace or deform the optical path that another optical signal takes and consequently alter its propagation [1] , [2] , [3] , [4] . Such an optomechanical effect permits optical signals to interact directly and can be implemented on an integrated device platform using only optically passive materials such as silicon and glass, circumventing the conventional need of electro-optical conversion or nonlinear optical materials [5] , [6] , [7] , [8] , [9] . Using high finesse optical cavities, optomechanical interaction can be resonantly enhanced. Research in cavity optomechanics exploits the dynamical interplay between the intra-cavity optical field and the mechanical motion of the device, leading to demonstrations of unprecedented phenomena including backaction cooling [10] , [11] , [12] , [13] , normal mode splitting [14] and optomechanically induced transparency [15] , [16] . Other than fundamental studies, a plethora of promising applications of cavity optomechanics, including tunable photonic filters and wavelength router [5] , [6] , wavelength conversion and switching [8] , [9] , radio-frequency optomechanical oscillators [17] , [18] and non-volatile optical memory [19] , have emerged. However, in the cavity optomechanical systems demonstrated so far, only one optical channel is available for both excitation and detection lasers to couple into the cavity. For example, in systems based on micro- and nanoscale cavities, optical coupling with the cavity is through either a single optical fiber [5] , [20] , [21] or an integrated waveguide [6] , [22] . Furthermore, in these systems, because the mechanical element is embedded inside the high finesse cavity, optomechanical effects can only be interrogated within extremely narrow bandwidths at the discrete resonance frequencies. These requirements impose a stringent limitation on the available spectral range to operate cavity optomechanical devices, thus limiting the prospect of practical applications. Should cavity optomechanics be integrated with other photonic devices, which may work at very different frequencies such as in a wavelength multiplexed system, a broad operation bandwidth would be necessary. We propose a multichannel scheme of cavity optomechanics with two waveguides that separate the mechanical element from the optical cavity. The first waveguide is denoted as the control that is used to couple a laser into the cavity to excite its resonance and generate optomechanical force. The mechanical element resides outside the cavity in the second signal waveguide so that its optomechanical motion can be readout over a broad wavelength range. When tuned to resonance, the cavity resonantly enhances the optical force on the mechanical element. Moving the mechanical element out of the optical cavity and adding the second waveguide has the following benefits: first, the mechanical device can be optimized without sacrificing the quality of the optical cavity; second, the thermo-optic effect that often plagues optomechanical effects becomes insignificant because the mechanical device is outside the cavity and the readout signal can be decoupled from the cavity resonance; third and more importantly, the freedom to use a readout wavelength in the signal waveguide over a broad band offers great flexibility for cavity optomechanics to be integrated with other nanophotonic devices to achieve advanced functionalities. Multichannel design of a cavity optomechanical device Our device is comprised of a micro-disk cavity coupled with a control and a signal waveguide, in the typical configuration of an add-drop filter as illustrated in Fig. 1a . A scanning electron microscope image of the actual device is shown in Fig. 1b . The control waveguide at the top couples with the micro-disk with a gap of 120 nm, providing the first channel to excite the resonance modes of the cavity. The second channel is through the signal waveguide at the bottom. In it, a small gap (50 nm) is created and a 22-μm long cantilevered waveguide is suspended from the substrate. The evanescent optical field of the micro-disk's resonance mode applies a gradient optical force on the signal waveguide and, inversely, the signal waveguide's motion also dispersively perturbs the cavity's resonance [20] , [22] . In contrast to the conventional phase sensitive detection method, which relies on the cavity resonance, the optomechanical motion of the signal waveguide is detected directly by monitoring the intensity of transmission. Previously it has been shown that this intensity detection scheme is inherently broadband; even an incoherent light source can be used to achieve high detection sensitivity [23] . To limit the number of resonance modes, the micro-disk is designed in an annular shape with a major and a minor radius of 10 and 5 μm, respectively. The measured transmission spectrum through the control waveguide and the coupling spectrum from the control to the signal waveguide (that is, the drop port transmission as in an add-drop filter) are shown in Fig. 1c , where each resonance mode is labeled with its radial and azimuthal mode order number as ( p , m ). Transverse-electric (TE) resonance modes with radial mode number from one to five can be observed in the spectra. In the transmission spectrum of the control waveguide, the cavity modes show varying extinction ratios because of the difference in their coupling efficiency with the waveguide mode. Among them, we focus on the TE mode (4, 89) that has the highest loaded quality factor Q of 5×10 4 (corresponding finesse is 561) and extinction ratio of more than 20 dB, indicating a nearly critical coupling condition. The inset of Fig. 1c shows the square of the transverse electric field component of the fourth-order radial mode, calculated with finite element method [24] . To detect the cantilevered signal waveguide's motion, the transmission of the signal waveguide is monitored using a laser with any wavelength that is different from the micro-disk's resonance (for example, at 1,555 nm in Fig. 1c ). To obtain a linear response to its motion, the fixed end of the waveguide is designed during patterning to offset laterally from the cantilevered end by 250 nm, causing a manageable addition of 3 dB insertion loss (see Supplementary Methods ). 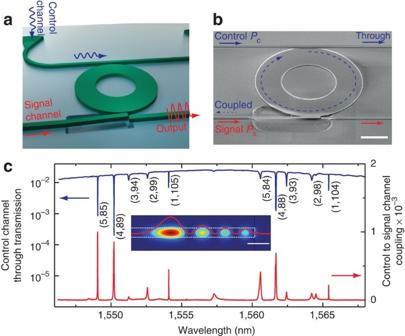Figure 1: A multichannel cavity optomechanical device. (a) Schematic illustration of the device, which features a micro-disk cavity coupled with a control and a signal channel waveguide. The key mechanical element is the cantilevered section in the signal waveguide whose motion can be detected over a broad bandwidth by measuring the optical transmission of the waveguide. (b) Scanning electron microscopy image of the device, highlighting the micro-disk (10 μm in radius) and the cantilever waveguide. Scale bar, 5 μm. (c) The measured spectra of the transmission through the control waveguide (blue trace, logarithmic scale, left axis) and the coupling from the control to the signal waveguide (red trace, linear scale, right axis), respectively. Inset: finite element simulation result showing the square of transverse electric field component and its profile (red overlay curve) of the fourth radial modes. The dashed box outlines the micro-disk. Scale bar, 0.5 μm. Figure 1: A multichannel cavity optomechanical device. ( a ) Schematic illustration of the device, which features a micro-disk cavity coupled with a control and a signal channel waveguide. The key mechanical element is the cantilevered section in the signal waveguide whose motion can be detected over a broad bandwidth by measuring the optical transmission of the waveguide. ( b ) Scanning electron microscopy image of the device, highlighting the micro-disk (10 μm in radius) and the cantilever waveguide. Scale bar, 5 μm. ( c ) The measured spectra of the transmission through the control waveguide (blue trace, logarithmic scale, left axis) and the coupling from the control to the signal waveguide (red trace, linear scale, right axis), respectively. Inset: finite element simulation result showing the square of transverse electric field component and its profile (red overlay curve) of the fourth radial modes. The dashed box outlines the micro-disk. Scale bar, 0.5 μm. Full size image We first demonstrate the actuation of the signal waveguide by exciting the resonance of the micro-disk from the control waveguide. The evanescent field of the circulating light in the micro-disk generates a gradient optical force on the signal waveguide [20] , [22] . This force is attractive toward the micro-disk and can be expressed as [22] : Here, x is the signal waveguide's lateral position (positive is in the direction away from the micro-disk), P in is the input optical power in the control waveguide. δ =( ω − ω c )/γ is the normalized detuning of the control laser frequency ω relative to the cavity resonance frequency ω c ( x ), which is dependent on the position of the signal waveguide. γ = γ 1 + γ 2 + γ i = ω c /2 Q is the total damping rate of the cavity including the coupling rate with the control and the signal waveguides γ 1 and γ 2 , respectively, and the cavity's intrinsic damping rate γ i . g ( x ) is the important optomechanical coupling coefficient, which under the perturbation approximation [20] , depends exponentially on the signal waveguide's displacement δx = x − x 0 and can be expressed as g ( x )=∂ ω c /∂ x=g 0 exp(−2 α δx) , where α is the evanescent field decay constant of the cavity resonance mode. In our device, the static value of g 0 for the TE mode (4,89) is experimentally determined to be 2π×π11.3 MHz nm −1 (see Supplementary Methods ) [25] . From equation (1), it is clear that when the control laser frequency is tuned to the cavity resonance ( δ 0 = δ ( x = x 0 )=0), the static optical force F c ( x 0 ) will be maximized, enhanced by the cavity power build-up factor. Modulating the input power P in will generate a time varying optical force on the cantilever waveguide to excite its mechanical resonance. 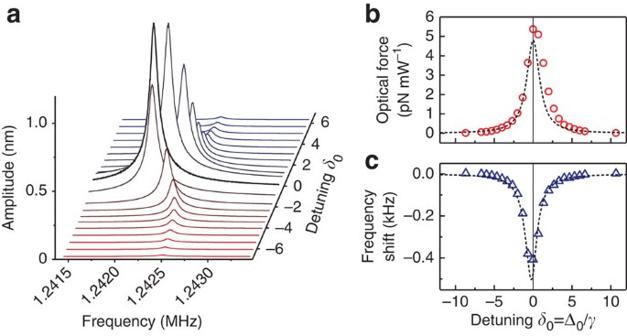Figure 2: Optical force and optical spring effect. (a) Small amplitude resonance response of the cantilevered signal waveguide driven by the control laser with constant power (alternating current (AC) power: 0.76 μW, DC power: 0.52 mW) and varying detuning. The vibration amplitude reaches maximum when the control laser is tuned to the cavity resonance. (b,c) Total attractive optical force on the signal waveguide and resonance frequency shift as a function of detuning. Black dashed lines show theoretical results (seeSupplementary Discussion). Figure 2a shows the measured small-amplitude mechanical response of the signal waveguide using a low modulated optical power (0.76 μW peak value) but varying detuning value δ 0 . The signal waveguide vibrates with a resonance frequency of 1.24 MHz and a quality factor Q m of 1.6×10 4 in vacuum. The resonance amplitude increases drastically when the detuning approaches zero. Figure 2b shows the calibrated measurement of the optical force (normalized to the input power) on the signal waveguide versus detuning values, demonstrating a resonant enhancement factor of more than 500 as expected from the theory (see Supplementary Methods for the force calibration procedure). In addition, the mechanical frequency of the signal waveguide also appears to depend on the detuning, as shown in Fig. 2c . This dependence is known as the optical spring effect from the linear variation of optical force with the device's position. In contrast to conventional cavity optomechanics in which the optical spring vanishes when the detuning is zero [26] , [27] , [28] , our result shows a maximal negative frequency shift near zero detuning, indicating the strongest negative optical spring. This distinction is because the optical force in our system is generated by the evanescent field outside the cavity, instead of the intra-cavity field. The observed phenomenon can be well explained theoretically as plotted with dashed lines in Fig. 2b,c and discussed in detail in the Supplementary Discussion . Figure 2: Optical force and optical spring effect. ( a ) Small amplitude resonance response of the cantilevered signal waveguide driven by the control laser with constant power (alternating current (AC) power: 0.76 μW, DC power: 0.52 mW) and varying detuning. The vibration amplitude reaches maximum when the control laser is tuned to the cavity resonance. ( b , c ) Total attractive optical force on the signal waveguide and resonance frequency shift as a function of detuning. Black dashed lines show theoretical results (see Supplementary Discussion ). Full size image Controllable optomechanical nonlinearity Cavity optomechanical devices are inherently nonlinear mechanical systems [29] because the optomechanical interaction involves the intra-cavity field, which depends nonlinearly on the mechanical elements' position. Exploiting the nonlinear dynamics in cavity optomechanical systems will be especially important to applications that need to operate the devices in the high-amplitude regime, such as optomechanical oscillators [17] , [18] and optomechanical memory [19] . As can be seen from equation (1), the optical force F c in our device is a nonlinear function of the signal waveguide's displacement δx = x − x 0 . The expression can be expanded near the static position x 0 to the higher orders of δx as F c ( x )= F c ( x 0 )+ k 1 δx + k 2 δx 2 + k 3 δx 3 + O ( δx 4 ). Here, k 1 is the force constant of the optical spring, k 2 and k 3 are the quadratic and cubic nonlinear force constants, respectively. The mechanical frequency of the signal waveguide is modified by the optical spring k 1 to be ω m 2 = ω m 0 2 − k 1 / m eff , where m eff is the effective mass of the fundamental mechanical resonance mode. The nonlinear components in the optical force induce mechanical nonlinearity with quadratic and cubic nonlinear coefficients given by: α 2 (=− k 2 / m eff ) and α 3 (=− k 3 / m eff ). In the small-amplitude regime, the nonlinear terms are insignificant and only the frequency down shift due to the optical spring k 1 can be observed as in Fig. 2 . When the signal waveguide's vibration is excited to large amplitude, the cubic nonlinear term becomes important and the signal waveguide vibrates as a nonlinear Duffing oscillator with bifurcation in its frequency response. In this regime, the quadratic term as a small correction to the Duffing nonlinearity is negligible [30] . The critical amplitude a c , at which the intrinsic mechanical nonlinearity becomes evident, is evaluated to be about 1μm using the expression (ref. 31 ), where L =22 μm is the length of the cantilever and Q m =1.6×10 4 is its mechanical Q factor. Such large amplitude cannot be reached in our device because the gap between the micro-disk and the signal waveguide is only 120 nm. However, the optomechanical contribution to the cubic coefficient α 3 is proportional to the optical power level (see Supplementary Discussion ). Hence, even at amplitude much lower than a c , with sufficient optical power strong optomechanical nonlinearity can be induced to dominate the device's mechanical response. To demonstrate the optomechanical nonlinearity, we apply a third laser, denoted as the tuning laser, with a static power level to the control waveguide. The magnitude of the induced optomechanical nonlinearity can be controlled by varying the power level and the frequency of the tuning laser. The result is shown in Fig. 3 . With the tuning laser power at as low as 100 μW (in the control waveguide), strong nonlinearity can be observed when the signal waveguide's vibration amplitude is above 50 nm, only one-twentieth of the mechanical critical amplitude a c . Most interestingly, the detuning of the tuning laser has a significant effect on the device's nonlinearity. 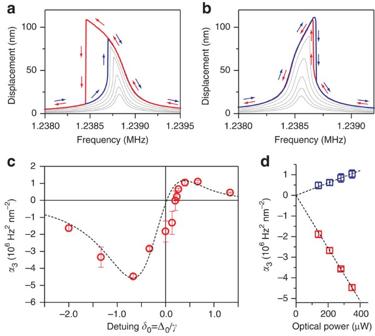Figure 3: Controllable optomechanical nonlinearity. (a,b) Amplitude-frequency response curves of the signal waveguide under increasing drive amplitude, measured with 350μW tuning laser red-detuned (a,δ0=−0.5) and blue-detuned (b,δ0=0.4) to the cavity resonance. The red and blue curves are obtained by sweeping the drive frequency downward and upward, respectively, and with the same modulation level. (c) The measured cubic (Duffing) nonlinear coefficientα3as a function of tuning laser detuning.α3can be controlled to be negative or positive by changing the detuning. Black dashed line shows the theoretical results with no free parameters, using only experimentally determined and numerically simulated values of the parameters. Error bars: s.d. from five measurements. (d) The measured valueα3for red (δ0=−0.67) and blue (δ0=0.67) detuned laser at various optical power of the applied tuning laser, showing a proportional dependence. Error bars: s.d., from five measurements. Figure 3a and b show the measured amplitude-frequency response when the modulation level of the control laser power is gradually increased (direct current (DC) power is constant at 80μW) and the tuning laser power is fixed at 350 μW. When the tuning laser is red-detuned to the cavity resonance ( Fig. 3a , δ 0 =−0.5), the response shows the softening nonlinearity of a typical Duffing oscillator with the characteristic amplitude jumps and the hysteresis effect when the actuation frequency is swept upward (blue trace) and downward (red trace), indicating that the cubic nonlinear coefficient α 3 is negative. The situation changes when the tuning laser is blue-detuned, the response instead shows hardening nonlinearity ( Fig. 3b , δ 0 =0.4), indicating a positive α 3 . From these measured response curves, the value of α 3 can be determined experimentally (see Supplementary Methods ) and the results for varying detuning δ 0 are plotted in Fig. 3c . It clearly shows that the cubic nonlinear coefficient is controlled by the tuning laser and its sign can be changed depending on the detuning. The maximal negative and positive values of α 3 are obtained experimentally with δ 0 equals −0.67 and 0.67, respectively. At blue detuning of δ 0 ~0.02, the value of α 3 vanishes and the cubic nonlinearity diminishes, allowing higher order nonlinearity to appear. The theoretical value of α 3 is also calculated using only experimentally determined and numerically simulated values of the parameters in equation (1) and plotted in Fig. 3c (see Supplementary Discussion for detailed theoretical analysis), in an excellent agreement with the experimental result. The deviation is attributed to the imprecision in determining the actual detuning value because of the thermal drift of the cavity resonance. Figure 3d shows that the value of α 3 is proportional to the power of the tuning laser for both softening (red) and hardening (blue) situations, as expected from theoretical analysis. The rich and completely controllable optomechanical nonlinearity in cavity optomechanics, demonstrated here for the first time, can be harnessed to explore nonlinear phenomena in nanomechanical oscillators [29] , including parametric amplification [32] , synchronization [33] and stochastic dynamics [34] , [35] . Figure 3: Controllable optomechanical nonlinearity. ( a , b ) Amplitude-frequency response curves of the signal waveguide under increasing drive amplitude, measured with 350μW tuning laser red-detuned ( a , δ 0 =−0.5) and blue-detuned ( b , δ 0 =0.4) to the cavity resonance. The red and blue curves are obtained by sweeping the drive frequency downward and upward, respectively, and with the same modulation level. ( c ) The measured cubic (Duffing) nonlinear coefficient α 3 as a function of tuning laser detuning. α 3 can be controlled to be negative or positive by changing the detuning. Black dashed line shows the theoretical results with no free parameters, using only experimentally determined and numerically simulated values of the parameters. Error bars: s.d. from five measurements. ( d ) The measured value α 3 for red ( δ 0 =−0.67) and blue ( δ 0 =0.67) detuned laser at various optical power of the applied tuning laser, showing a proportional dependence. Error bars: s.d., from five measurements. Full size image Optomechanical Signal Amplification In cavity optomechanics, by leveraging the enhancement from both the optical and mechanical resonances, a low-power optical signal can be used to modulate a high-power optical signal via their enhanced optomechanical interaction, making it possible to achieve a net signal gain at the modulation frequency. Such a mechanical means of signal amplification is analogous to the principles of electromechanical relays or electronic transistors ( Fig. 4a ) and has found important applications [36] , [37] . In addition, our multichannel design of cavity optomechanics features a broadband transmission in the signal waveguide, making wavelength multiplexing possible. In our device, the signal gain factor (GF) is defined as the ratio between the alternating current (AC) optical power input to the control waveguide and the modulated output power from the signal waveguide. 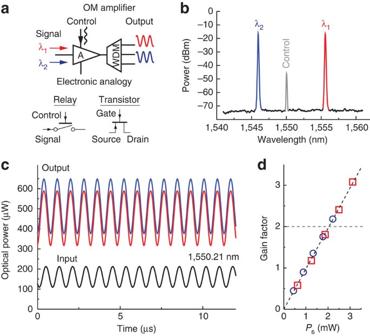Figure 4: All-optical signal amplification and wavelength multiplexing. (a) The principle of optomechanical amplification is analogous to that of electromechanical relays or electronic transistors. A small signal in the control waveguide (or gate) can be used to modulate a large signal in the signal waveguide (or source to drain) to achieve a signal gain. Wavelength multiplexing can also be achieved. (b) Optical spectrum measured at the output of the signal waveguide, showing signals at two wavelengths and the leaked control. (c) Time domain traces of the input (black) and output signals at two different wavelengths (blue: 1,546.12 nm and red: 1,555.75 nm), showing the input signal is amplified by a gain factor of three at the output. One output trace (blue) is intentionally shifted upward for clarity. (d) The gain factor is proportional to the optical power in the signal waveguide but independent of the signal wavelength (blue: 1,546.12 nm and red: 1,555.75 nm). A gain factor of two can be achieved with a signal power of only 2 mW. At the mechanical resonance frequency, GF is maximized and given by Figure 4: All-optical signal amplification and wavelength multiplexing. ( a ) The principle of optomechanical amplification is analogous to that of electromechanical relays or electronic transistors. A small signal in the control waveguide (or gate) can be used to modulate a large signal in the signal waveguide (or source to drain) to achieve a signal gain. Wavelength multiplexing can also be achieved. ( b ) Optical spectrum measured at the output of the signal waveguide, showing signals at two wavelengths and the leaked control. ( c ) Time domain traces of the input (black) and output signals at two different wavelengths (blue: 1,546.12 nm and red: 1,555.75 nm), showing the input signal is amplified by a gain factor of three at the output. One output trace (blue) is intentionally shifted upward for clarity. ( d ) The gain factor is proportional to the optical power in the signal waveguide but independent of the signal wavelength (blue: 1,546.12 nm and red: 1,555.75 nm). A gain factor of two can be achieved with a signal power of only 2 mW. Full size image Here, ∂ T s /∂ x is the response of the signal channel's transmission to the lateral motion of the cantilever waveguide, ∂ F c /∂ P c is the efficiency of optical force generation, which is enhanced by the cavity finesse as demonstrated in Fig. 2 . Although in principle arbitrarily large GF can be attained with sufficient signal power P s as GF is proportional to P s , in practice the maximal GF is limited by the power handling capability of the device. The high finesse of the micro-disk cavity and the high mechanical quality factor Q m and compliance (1/ k m ) of the cantilevered waveguide allows a high gain value to be attained with a low signal power P s . To demonstrate the principles of optomechanical amplification of radio-frequency signal and wavelength multiplexing with our device, two continuous wave (CW) lasers were input to the signal waveguide and the control laser was modulated at the mechanical resonance frequency. Figure 4b shows the optical spectra at the output of the signal waveguide, showing the two optical signals at wavelength λ 1 and λ 2 , which can be freely selected over a broad spectral range as long as the cavity resonance wavelengths are avoided. Also seen in Fig. 4b is the leaked control laser with 30 dB lower power than the signal lasers because the micro-disk also acts as a filter. A standard wavelength division-multiplexing filter is used to separate the two signals at wavelengths λ 1 and λ 2 . Figure 4c shows the time domain traces of the input modulation signal (DC power 170 μW at 1,550.21 nm) at the control waveguide and two output signals (DC power 450 μW at 1,546.12 and 1,555.75 nm) from the signal waveguide, modulated at the mechanical resonance frequency of 1.24 MHz. The result shows that the modulated amplitude of the input signal is amplified by a factor of three in the output signal. Because of the broadband signal waveguide, this GF is independent of the signal wavelength so the device is suited to optical systems using wavelength multiplexing. The GF increases proportionally with the input signal power P s and is consistent for the two different signal wavelengths, as shown in Fig. 4d . Similar silicon micro-disk cavity with quality factor as high as 3 million has been reported in the literature [38] so it is possible to achieve even higher GF with a much lower power level. Although the operation speed of the device currently is limited by the relatively low mechanical frequency of the cantilevered signal waveguide, it is feasible to improve the mechanical frequency to the hundreds of megahertz range [39] , [40] , making it suited for radio-frequency (RF) photonics applications. Recently, micro- and nanoscale mechanical switches and relays have been revisited for their potential in integrated circuits for low power computation [41] and for harsh environment applications [42] . Optomechanical devices also provide unique attributes that are unattainable with conventional optical devices, such as the all-optical signal amplification demonstrated here and the ability to be reconfigured and re-programmed [6] , [20] , [43] . The broad optical bandwidth enabled by the new multichannel configuration offers great flexibility for cavity optomechanics to be integrated at a higher level, allowing their remarkable properties to be applied in cohorts with conventional photonic systems for optical and RF communications. Device The devices are fabricated on commercial SOI wafers (SOITEC) with 220 nm silicon layer and 3 μm buried oxide, using standard electron beam lithography and plasma dry etching processes. The cantilevered section of the signal waveguide is released from the substrate by wet etching the buried oxide layer through a photoresist mask patterned by photolithography. Critical point drying is used to prevent the collapsing of the cantilevered waveguide caused by the viscous dragging effect during etchant solution evaporation. The released section of the signal waveguide is 22 μm long, 420 nm wide with a mechanical spring constant of 69.4 mN m −1 . With a gap of 50 nm and a lateral offset of 250 nm between the cantilevered end and the receiving end, the signal waveguide has an estimated total insertion loss of 7.8 dB. Measurement scheme and device A schematic of the measurement setup is shown in Supplementary Figure S8 . The control, signal and tuning lasers are coupled into the device by aligning a linear array of single-mode fibers, spaced 250μm and mounted on a V-groove (OZ optics) chip, to the integrated grating couplers on the device. Each fiber to grating coupler interface has a typical coupling efficiency of 15%. All the power values mentioned in the manuscript refer to the power in the waveguide immediately after the coupler and are carefully calibrated and monitored. To achieve high mechanical quality factor, the measurements are conducted in a vacuum chamber with pressure of 2×10 −4 Torr. A microscope image of the device that is measured during the experiment is shown in Supplementary Figure S9 . How to cite this article: Li, H. et al . Multichannel cavity optomechanics for all-optical amplification of radio frequency signals. Nat. Commun. 3:1091 doi: 10.1038/ncomms2073 (2012).